An intestinal commensal symbiosis factor controls neuroinflammation via TLR2-mediated CD39 signalling The mammalian immune system constitutively senses vast quantities of commensal bacteria and their products through pattern recognition receptors, yet excessive immune reactivity is prevented under homeostasis. The intestinal microbiome can influence host susceptibility to extra-intestinal autoimmune disorders. Here we report that polysaccharide A (PSA), a symbiosis factor for the human intestinal commensal Bacteroides fragilis , protects against central nervous system demyelination and inflammation during experimental autoimmune encephalomyelitis (EAE), an animal model for multiple sclerosis, through Toll-like receptor 2 (TLR2). TLR2 mediates tissue-specific expansion of a critical regulatory CD39 + CD4 T-cell subset by PSA. Ablation of CD39 signalling abrogates PSA control of EAE manifestations and inflammatory cytokine responses. Further, CD39 confers immune-regulatory phenotypes to total CD4 T cells and Foxp3 + CD4 Tregs. Importantly, CD39-deficient CD4 T cells show an enhanced capability to drive EAE progression. Our results demonstrate the therapeutic potential and underlying mechanism by which an intestinal symbiont product modulates CNS-targeted demyelination. The skin and mucosal surfaces of humans are colonized by a wide variety of commensal microorganisms that outnumber human somatic cells [1] . The gastrointestinal tract harbours the greatest quantity and diversity of microorganisms. Traditionally appreciated for its function to facilitate metabolism and nutrient intake, intestinal microbiome has now been intensively studied for its role in maintaining host immune homeostasis [2] , [3] , [4] , [5] . The composition of intestine microbiota, or enterotype, influences host predisposition to autoimmune disorders, affecting tissue sites proximal and distal to the intestine [6] , [7] , [8] , [9] , [10] , [11] . Experimental autoimmune encephalomyelitis (EAE) is an animal model of human multiple sclerosis where self-reactive immune pathology targets the central nervous system (CNS). Although colonization of germ-free mice with segmented filamentous bacteria increases susceptibility to EAE, oral administration with Bacteroides fragilis , Bifidobacterium animalis and other probiotic mixtures have been shown to prevent EAE development [12] , [13] , [14] , [15] , [16] . These studies associated different commensal strains with opposite outcomes of CNS autoimmunity. Commensal bacteria can be characterized as symbionts or pathobionts, depending on the survival strategies employed. Symbionts live in a lifelong mutualistic pattern with the host, whereas pathobionts are often opportunistic pathogens [5] . To facilitate co-existence, symbionts must limit aggressive immune attacks or induce immune tolerance by using some microbial products as symbiosis factors. In this context, polysaccharide A (PSA) produced by the human intestinal symbiont B. fragilis has been identified as a model molecule that elicits beneficial immune responses for both commensals and host. B. fragilis lacking PSA have defective mucosal colonization due to the inability to restrain Th17 responses [17] . Initially found to direct host adaptive immunity maturation, PSA then reveals its capability of resolving autoimmunity [18] , [19] . Oral treatment with PSA prevents murine experimental colitis by inducing IL-10 + Foxp3 + regulatory T cells (Tregs) [20] . Notably, PSA also suppresses CNS inflammation during murine EAE, operational through interleukin (IL)-10 and CD103 + dendritic cells (DCs) [21] . The precise signal by which PSA imparts on the adaptive immune cells, particularly the CD4 + T cells, to prevent disease progression remains uncertain. Microbial ligands are detected by host innate immunity as microbe-associated molecular patterns. Sensing of microbial ligands by Toll-like receptors (TLRs) can mobilize innate immunity and subsequently activate adaptive immunity, leading to the host exclusion of microbes [22] . PSA, however, represents a reverse example where TLR detection of microbial ligand promotes the co-existence of symbionts with the host. TLR2 signals on CD4 + T cells are crucial for PSA elicitation of immunologic tolerance towards B. fragilis intestinal colonization [17] . Further, although many other microbial ligands sensed by TLRs act as adjuvants to exacerbate autoimmunity, detection of PSA by TLR2 resolves intestinal inflammation [20] , [23] , [24] . Our previous study has shown that oral treatment with B. fragilis PSA prevents murine EAE both prophylactically and therapeutically [21] . In this study, we demonstrate that TLR2 signalling is essential for PSA-mediated modulation of CNS immune pathology. The expansion of CD39 + CD4 + T cells downstream TLR2 is responsible for PSA-mediated immune regulation. CD39 defines regulatory phenotypes in CD4 T cells irrespective of Foxp3 co-expression and is essential for the protective function of PSA during CD4 + T cell-driven neuroinflammation. B. fragilis PSA controls CNS inflammation via TLR2 To evaluate whether TLR2 is required for PSA regulation of CNS inflammatory disease, wild-type (WT) or TLR2 KO mice were given oral prophylactic treatment with PSA or PBS during EAE. Consistent with previous results, treatment with PSA in WT mice delayed the clinical onset and progression of EAE, as reflected by the clinic curve and cumulative score. The protective effects were abrogated in TLR2 KO mice. At basal level, PBS-treated WT and TLR2 KO mice developed comparable severity of EAE ( Fig. 1a,b ). Histological assays confirmed the clinical results. Haematoxylin and eosin (H&E) staining ( Fig. 1c , first and third columns) revealed that PSA inhibited the robust lymphocyte infiltration into the CNS (spinal cord and brain) in WT mice. This inhibitory function of PSA was abrogated in TLR2 KO mice. Lymphocytic influx leads to demyelination in EAE. As Luxol fast blue staining ( Fig. 1c , second column) showed, although PSA reduced demyelination lesions of the spinal cord in WT mice, this effect was not observed in TLR2 KO mice. Oral therapeutic treatment with PSA also protects against EAE via TLR2 ( Supplementary Fig. 1 ). 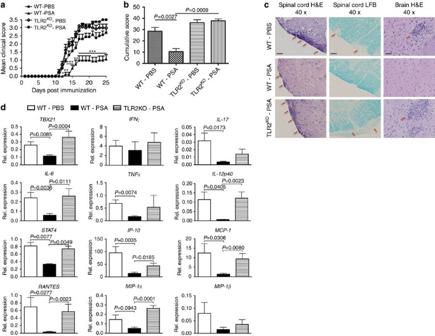Figure 1: Oral treatment withB. fragilisPSA protects against murine EAE in a TLR2-dependent manner. WT and TLR2KOmice on C57BL/6 background were prophylactically treated with 100 μg of purifiedB. fragilisPSA or PBS as control by oral gavage every 3 days. Treatment was initiated 6 days before optimal active EAE induction (subcutaneous injection with MOG35–55peptide plus two doses of intraperitoneal injection with pertussis toxin) and terminated 9 days after disease induction. (a) EAE clinic scores were monitored till day 25. Depicted are the combined results of two independent experiments (n=8, per group). Mean±s.e.m. scores are shown. *P<0.05; **P<0.01; ***P<0.001 (Kruskal–Wallis test of all groups). (b) Cumulative scores were derived fromaas the sum of clinic scores divided by the number of mice per group. Mean±s.e.m. scores are shown.P-value was calculated by Mann–WhitneyU-test. (c) Histological analyses show transversal sections of spinal cords stained with H&E and Luxol fast blue (LFB), and sections of brain stems stained with H&E. H&E stain targeted nucleated cells (red arrows point at the clusters of infiltrating lymphocytes); LFB stain targeted myelin (red arrows point at the demyelination spots). Depicted are representative pictures (magnification × 40) from the indicated EAE-induced groups: PBS-treated WT mice, PSA-treated WT mice and PSA-treated TLR2KOmice. All samples were collected (n=4 sections per mouse,n=3 mice per group) at the peak of disease. Images in each row are the same treatment group, and in each column are the same staining method. Scale bars, 100 μm. (d) Brains of PBS or PSA-treated EAE-induced WT mice or PSA-treated EAE-induced TLR2KOmice were harvested at the onset stage of the disease. Relative expression of transcription factors (Tbx21,Stat4), cytokines (interferon-γ, IL-17, IL-6, TNFα, IL-12p40) and chemokines (IP-10, MCP-1, Rantes, MIP-1α, MIP-1β) were measured by quantitative RT–PCR. Mean±s.e.m. mRNA relative expression from two independent experiments is shown.P-value was calculated by two-tailed Student’st-test (n=5–12 for each group). Figure 1: Oral treatment with B. fragilis PSA protects against murine EAE in a TLR2-dependent manner. WT and TLR2 KO mice on C57BL/6 background were prophylactically treated with 100 μg of purified B. fragilis PSA or PBS as control by oral gavage every 3 days. Treatment was initiated 6 days before optimal active EAE induction (subcutaneous injection with MOG 35–55 peptide plus two doses of intraperitoneal injection with pertussis toxin) and terminated 9 days after disease induction. ( a ) EAE clinic scores were monitored till day 25. Depicted are the combined results of two independent experiments ( n =8, per group). Mean±s.e.m. scores are shown. * P <0.05; ** P <0.01; *** P <0.001 (Kruskal–Wallis test of all groups). ( b ) Cumulative scores were derived from a as the sum of clinic scores divided by the number of mice per group. Mean±s.e.m. scores are shown. P -value was calculated by Mann–Whitney U -test. ( c ) Histological analyses show transversal sections of spinal cords stained with H&E and Luxol fast blue (LFB), and sections of brain stems stained with H&E. H&E stain targeted nucleated cells (red arrows point at the clusters of infiltrating lymphocytes); LFB stain targeted myelin (red arrows point at the demyelination spots). Depicted are representative pictures (magnification × 40) from the indicated EAE-induced groups: PBS-treated WT mice, PSA-treated WT mice and PSA-treated TLR2 KO mice. All samples were collected ( n =4 sections per mouse, n =3 mice per group) at the peak of disease. Images in each row are the same treatment group, and in each column are the same staining method. Scale bars, 100 μm. ( d ) Brains of PBS or PSA-treated EAE-induced WT mice or PSA-treated EAE-induced TLR2 KO mice were harvested at the onset stage of the disease. Relative expression of transcription factors ( Tbx21 , Stat4 ), cytokines (interferon-γ, IL-17, IL-6, TNFα, IL-12p40) and chemokines (IP-10, MCP-1, Rantes, MIP-1α, MIP-1β) were measured by quantitative RT–PCR. Mean±s.e.m. mRNA relative expression from two independent experiments is shown. P -value was calculated by two-tailed Student’s t -test ( n =5–12 for each group). Full size image CNS inflammation is the hallmark of both human multiple sclerosis and murine EAE [25] , [26] . To investigate whether PSA restricts CNS inflammation via TLR2, transcriptional levels of genes in the brain were compared for PSA versus PBS-treated WT mice and PSA-treated WT versus TLR2 KO mice ( Fig. 1d ). PSA downregulated multiple genes through TLR2 that encode for (1) transcription factors Tbx21 ( T-bet ) and Stat4 , which govern Th1 cell development; (2) pro-inflammatory cytokines IL-17, IL-6 and IL-12p40, which mediate Th1/Th17 as well as tumour necrosis factor-α (TNFα); (3) chemokines IP-10 (CXCL10), MCP-1 (CCL2), Rantes (CCL5), MIP-1α (CCL3) and MIP-1β (CCL4), which are attractants for T cell, macrophages and monocytes. In TLR2 KO mice, PSA failed to restrict or might exacerbate the expression of inflammation-related genes. The expression trend of chemokines in the CNS corroborated the histological visualization by H&E staining. Taken together, these results demonstrated that TLR2 is required for B. fragilis PSA control of CNS inflammation during EAE. PSA triggers specific signal on CD4 T cells via TLR2 CD4 + T cells are the primary immune population that drives EAE pathogenesis [25] . Cervical lymph nodes (CLNs) are important anatomical sites for immune cells draining to the CNS during autoimmunity [27] . Flow cytometric profiles of CLN CD4 + T cells were compared for PSA- or PBS-treated WT or TLR2 KO mice by mean fluorescence intensity (MFI) ( Fig. 2 ). A pool of CD4 + T-cell lineage and functional markers was included. CD39 was identified as a significant PSA- and TLR2-specific signal, which is correlated by comparing positive subset frequencies in Supplementary Fig. 2 . Both CD39 and CD73 are classified as ectonucleotidase, whose main function is to coordinate the conversion of extracellular ATP/ADP into adenosine [28] , [29] . CD73 signal on CLN CD4 + T cells, however, did not appear to be regulated through PSA/TLR2 axis ( Supplementary Fig. 3 ). 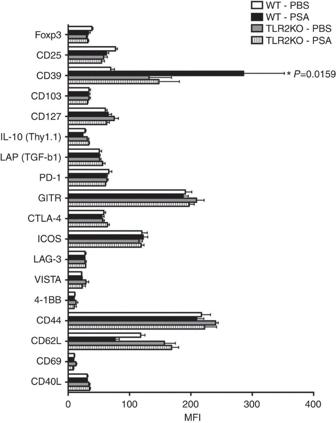Figure 2: PSA triggers specific signal on CD4 T cells via TLR2 under inflammatory conditions. WT and TLR2KOmice on IL-10 Thy1.1 reporter strain (10BiT) background were orally gavaged with PSA or PBS, and induced with optimal active EAE as inFig. 1asetting. At the peak of disease, total leukocytes were isolated from CLNs. Flow cytometry analysis was performed to identify the specific CD4 T-cell marker(s) triggered by PSA in a TLR2-dependent manner. CD4 T cells were pre-gated and MFI was used to measure the expression level of the indicated markers. Mean±s.e.m. MFI values were compared between PSA- or PBS-treated WT or TLR2KOmice. Depicted are representative results from two independent experiments (n=4 for each group).P-value was calculated by one-way analysis of variance test. Figure 2: PSA triggers specific signal on CD4 T cells via TLR2 under inflammatory conditions. WT and TLR2 KO mice on IL-10 Thy1.1 reporter strain (10BiT) background were orally gavaged with PSA or PBS, and induced with optimal active EAE as in Fig. 1a setting. At the peak of disease, total leukocytes were isolated from CLNs. Flow cytometry analysis was performed to identify the specific CD4 T-cell marker(s) triggered by PSA in a TLR2-dependent manner. CD4 T cells were pre-gated and MFI was used to measure the expression level of the indicated markers. Mean±s.e.m. MFI values were compared between PSA- or PBS-treated WT or TLR2 KO mice. Depicted are representative results from two independent experiments ( n =4 for each group). P -value was calculated by one-way analysis of variance test. Full size image PSA expands CD39 + CD4 T cells via TLR2 at specific tissues To further characterize in vivo regulation of CD39 signal on CD4 T cells, we examined the frequencies of CD39 + subset within CD4 T cells in EAE-induced WT or TLR2 KO mice orally treated with PBS or PSA. Consistent with MFI trends in Fig. 2 , representative histograms showed that PSA stimulated CD39 signal on CD4 T cells via TLR2 at both CLNs ( Fig. 3a ) and mesenteric lymph nodes (MLNs) ( Fig. 3b ). To determine whether the TLR2-dependent PSA expansion of CD39 + CD4 T cell subsets is local or systemic, frequencies of CD39 + subsets among CD4 T cells were quantified for CLNs, MLNs, spleen, whole blood ( Fig. 3c ) and immunization draining lymph nodes (DLNs) ( Supplementary Fig. 4 ). Of these tissue sites, only CLNs and MLNs displayed TLR2-dependent PSA upregulation of CD39 + CD4 T cells. CD39 + frequencies within splenic CD4 T cells were not affected. CD39 + frequencies within blood and DLN CD4 T cells were downregulated with PSA treatment. PSA does not significantly alter CD4 T cell-derived CD39 signals via TLR2 in naive mice ( Supplementary Fig. 5 ). Thus, the TLR2-dependent PSA expansion of CD39 + CD4 T cells during EAE is localized. Among lymphocytes, CD39 is expressed on both CD4 + T cells and B cells [29] . To investigate whether B cell-derived CD39 signal is concomitantly regulated by PSA/TLR2 axis at the affected sites, CD39 + frequencies within CD19 + B cells were quantified for CLNs and MLNs ( Fig. 3d ). Although CD19 + B cells showed higher basal level CD39 + frequencies compared with CD4 + T cells, PSA treatment did not significantly alter CD39 + frequencies within B cells. In vitro , PSA stimulated CD39 signals on CD4 T cells through DCs ( Supplementary Fig. 6A–C ). In summary, these results show that TLR2-dependent PSA-mediated enhancement of CD39 signal is both CD4 T cell-specific and tissue site-specific. 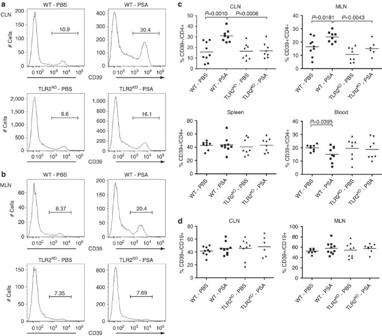Figure 3: TLR2-dependent PSA expansion of CD39+CD4 T cells is tissue site specific. WT and TLR2KOmice were treated with the same regimen as described inFig. 1asetting. At the peak of disease, total leukocytes were isolated from CLNs, MLNs, spleen and whole blood, and flow cytometry analysis was performed. Oral PSA administration stimulates CD39 expression on CD4 T cells via TLR2 at both (a) CLNs and (b) MLNs. CD4 T cells were pre-gated and CD39 expression level was measured inaandb. Depicted are the typical histograms for each indicated treatment group from two independent experiments (n=3–10, per group). (c) TLR2-dependent PSA induction of CD39 signal on CD4 T cells is restricted to CLNs and MLNs. Frequencies of CD39+subsets among CD4 T cells were quantified for the indicated tissue sites. Depicted are combined representative results of two independent experiments (n=6–10, per group).P-value was calculated by two-tailed Student’st-test. (d) PSA does not influence CD39 signal on CD19 B cells. Frequencies of CD39+subsets among CD19 B cells were quantified for both CLNs and MLNs. Combined representative results of two experiments are shown (n=6–10, per group). Figure 3: TLR2-dependent PSA expansion of CD39 + CD4 T cells is tissue site specific. WT and TLR2 KO mice were treated with the same regimen as described in Fig. 1a setting. At the peak of disease, total leukocytes were isolated from CLNs, MLNs, spleen and whole blood, and flow cytometry analysis was performed. Oral PSA administration stimulates CD39 expression on CD4 T cells via TLR2 at both ( a ) CLNs and ( b ) MLNs. CD4 T cells were pre-gated and CD39 expression level was measured in a and b . Depicted are the typical histograms for each indicated treatment group from two independent experiments ( n =3–10, per group). ( c ) TLR2-dependent PSA induction of CD39 signal on CD4 T cells is restricted to CLNs and MLNs. Frequencies of CD39 + subsets among CD4 T cells were quantified for the indicated tissue sites. Depicted are combined representative results of two independent experiments ( n =6–10, per group). P -value was calculated by two-tailed Student’s t -test. ( d ) PSA does not influence CD39 signal on CD19 B cells. Frequencies of CD39 + subsets among CD19 B cells were quantified for both CLNs and MLNs. Combined representative results of two experiments are shown ( n =6–10, per group). Full size image Phenotyping CLN-sourced CD39 + versus CD39 − CD4 T cells The phenotype of CD39 + CD4 T cells at inflammatory sites is not well understood. As PSA robustly stimulates CD39 + CD4 T cells at specific tissue sites during EAE, our study offers the opportunity to examine differences between inflammatory-state CD39 + and CD39 − CD4 T cells. CLNs were harvested from PSA-treated EAE-affected mice. Total CD4 + T cells were gated into CD39 + and CD39 − subsets and phenotyped by flow cytometry. The expression level of each individual marker was described by both histograms ( Fig. 4a ) and MFI ( Fig. 4b ). We found that the CD39 + CD4 T-cell subset, as compared with the CD39 − CD4 T-cell subset, expressed remarkably higher levels of IL-10 and significantly higher levels of latency-associated peptide, denoting tumour growth factor-β production. As for surface immune-regulatory markers, the CD39 + CD4 T-cell subset exhibited significantly higher levels of programmed death-1 (PD-1), glucocorticoid-induced tumour necrosis factor receptor-related gene ( GITR ), cytotoxic T-lymphocyte antigen 4 (CTLA-4), inducible T-cell costimulator (ICOS) and relatively higher expression of lymphocyte activation gene-3 ( LAG-3 ) and V-domain Ig suppressor of T-cell activation (VISTA). PD-1, GITR, CTLA-4, ICOS and LAG-3 are all co-inhibitory molecules with known ligands [30] , [31] , [32] ; VISTA is a co-inhibitory molecule with as yet no recognized ligand(s) [33] . Conversely, 4-1BB (CDw137), a co-stimulatory molecule, was noted at lower levels on the CD39 + CD4 T-cell subset [34] . 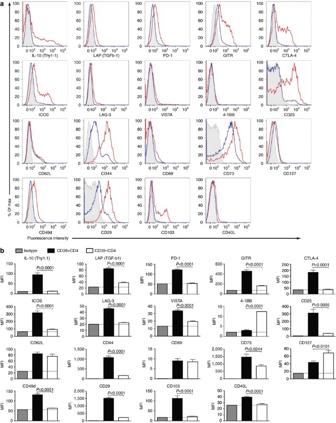Figure 4: Phenotyping CLN-sourced CD39+versus CD39−CD4 T cells. CLNs were harvested from PSA-gavaged EAE-induced mice (day 18 post EAE induction). Total leukocytes were isolated and analysed by flow cytometry. (a) CD39+CD4 T cells display elevated regulatory signatures as compared with CD39−CD4 T cells. CD39+and CD39-CD4 T-cell populations were analysed for the expression of each indicated marker. Depicted are the representative histograms for individual analysis from two independent experiments (n=4–5, per group). Red line, CD39+CD4 T cells; blue line, CD39−CD4 T cells; grey shade, isotype. (b) For each analysis ina, mean±s.e.m. MFI values were quantified. Black, CD39+CD4 T cells; white, CD39−CD4 T cells; grey, corresponding isotype for each indicated marker.P-value was calculated by two-tailed Student’st-test (n=4–5 for each group). Figure 4: Phenotyping CLN-sourced CD39 + versus CD39 − CD4 T cells. CLNs were harvested from PSA-gavaged EAE-induced mice (day 18 post EAE induction). Total leukocytes were isolated and analysed by flow cytometry. ( a ) CD39 + CD4 T cells display elevated regulatory signatures as compared with CD39 − CD4 T cells. CD39 + and CD39 - CD4 T-cell populations were analysed for the expression of each indicated marker. Depicted are the representative histograms for individual analysis from two independent experiments ( n =4–5, per group). Red line, CD39 + CD4 T cells; blue line, CD39 − CD4 T cells; grey shade, isotype. ( b ) For each analysis in a , mean±s.e.m. MFI values were quantified. Black, CD39 + CD4 T cells; white, CD39 − CD4 T cells; grey, corresponding isotype for each indicated marker. P -value was calculated by two-tailed Student’s t -test ( n =4–5 for each group). Full size image The expression of CD25 and CD44 positively correlated with CD39 in CD4 T cells, whereas CD62L and CD69 did not. Moreover, CD40L (CD154) expression was enriched within CD39 + CD4 T cells. These, in general, indicate that CD39 + CD4 T cell is an activated subset responsive to PSA exposure. CD39 + CD4 T-cell subset expressed remarkably higher CD49d and CD29 compared with CD39 − CD4 T-cell subset. CD49d (α4 integrin) and CD29 (β1 integrin) form very late antigen-4, a vital CNS-homing marker [35] . Increased level of CD73 was seen in CD39 + as opposed to CD39 − CD4 T-cell subset. CD39 + CD4 T-cell subset expressed relatively lower CD127 but remarkably higher CD103. CD127 (IL-7Rα) is downregulated on Treg cells [36] . CD103 (αE integrin) is mostly expressed by IELs but also by a subset of Tregs [37] . Collectively, CD39 + CD4 T cell is phenotyped as a regulatory subset with abundant expression of multiple immune-suppressive molecules. The regulatory phenotype of CD39 + CD4 T-cell subset was not confined to either tissue sites or treatment, as CD39 + CD4 T cell derived from other tissues or treatment groups displayed similar phenotypic pattern ( Supplementary Fig. 7 ). CD39 defines regulatory phenotypes regardless of Foxp3 Delineation of murine CD4 T cells by CD39 and Foxp3 revealed four populations: CD39 + Foxp3 + , CD39 − Foxp3 + , CD39 + Foxp3 − and CD39 − Foxp3 − ( Supplementary Fig. 8A ). To determine whether CD39 could confer regulatory phenotypes on its own, we further profiled CD39 + versus CD39 − Foxp3 + CD4 Treg ( Supplementary Fig. 8B ) and Foxp3 − CD4 Teff ( Supplementary Fig. 8C ) subsets sourced from CLNs of PSA-treated EAE-affected mice. The same markers as in Fig. 4 were used and quantified by MFI values. CD39 defined a similar expression profile of markers in Foxp3 + CD4 Tregs as in total CD4 T cells with exception to VISTA, CD40L and CD127 ( Supplementary Fig. 8B ). Further, CD39 defined a similar expression profile in Foxp3 − CD4 Teffs excluding VISTA, CD73, CD127 and CD40L ( Supplementary Fig. 8C ). Collectively, these data demonstrate that CD39 expression in response to PSA treatment is associated with multiple immune-suppressive features independent of Foxp3 co-expression. CD39 is essential for PSA-mediated immunoregulation in EAE To investigate the requirement for CD39 signalling in PSA-mediated suppression of CNS inflammation, WT or CD39 KO mice were orally gavaged with PSA before and after the induction of sub-optimal active EAE. CD39 deficiency abrogated the immune-regulatory function of PSA ( Fig. 5a,b ). WT and CD39 KO mice developed similar basal levels of EAE ( Supplementary Fig. 9 ). The similar clinic trend was observed in optimal EAE ( Supplementary Fig. 10 ). The clinic results in Fig. 5a,b were confirmed by histological assays. PSA-mediated suppression of lymphocyte influx and demyelinating lesions in the CNS was prominent in WT mice but diminished in CD39 KO mice ( Fig. 5c ). CD39 is required for PSA control of both neural and systemic inflammation during EAE ( Supplementary Fig. 11 ). PSA-treated WT mice exhibited lower T-cell activation levels than did PSA-treated CD39 KO mice. The trend was evident at CLN and also seen at MLN, but not at spleen or whole blood ( Fig. 5d ), correlating with the PSA-mediated site-specific expansion of CD39 + CD4 T cells. 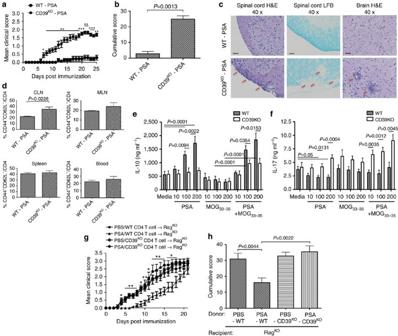Figure 5: CD39 signalling is essential for PSA-mediated immunoregulation during murine EAE. WT and CD39KOC57BL/6 mice were treated with PSA as inFig. 1aand induced sub-optimal active EAE. (a) EAE was monitored till day 25. Mean±s.e.m. scores typical of two independent experiments are shown (n=8, per group). *P<0.05; **P<0.01; ***P<0.001. (b) Mean±s.e.m. cumulative scores were calculated from (a). (c) H&E and Luxol fast blue (LFB) staining was performed same as inFig. 1c. Depicted are typical pictures (magnification × 40) from EAE-induced PSA-treated WT or CD39KOmice. All samples were collected (n=4 sections per mouse,n=3 mice per group) at the peak of disease. Scale bars, 100 μm. (d) Tissues were collected at the onset of EAE and flow cytometric analysis of cells was performed. Mean±s.e.m. frequencies of activated subsets within total CD4 T cells were compared for the indicated sites (n=4). (e,f) Total splenocytes were obtained from WT or CD39KOmice treated as inaon day 14 of EAE induction and culturedin vitrowith PSA, MOG35–55peptide, or a combination of both at escalating doses (10, 100 or 200 μg ml−1of each). Supernatants were collected 48 h after culture. IL-10 (e) and IL-17A (f) were measured by ELISA. Mean±s.e.m. results are combined from two experiments (n=3-4). (g) RagKOrecipient mice were reconstituted with splenic CD4 T cells from day 14 EAE-induced WT and CD39KOmice treated with PSA as inaor PBS. Two weeks later, optimal active EAE was introduced into recipients. EAE was monitored till day 21. Mean±s.e.m. scores representative of two experiments are shown (n=6–8, per group). *P<0.05; **P<0.01. (h) Mean±s.e.m. cumulative scores were derived fromg.P-value was calculated by Mann–WhitneyU-test ina,bandh, by two-tailed Student’st-test ind,eandf, and by Kruskal–Wallis test ing. Figure 5: CD39 signalling is essential for PSA-mediated immunoregulation during murine EAE. WT and CD39 KO C57BL/6 mice were treated with PSA as in Fig. 1a and induced sub-optimal active EAE. ( a ) EAE was monitored till day 25. Mean±s.e.m. scores typical of two independent experiments are shown ( n =8, per group). * P <0.05; ** P <0.01; *** P <0.001. ( b ) Mean±s.e.m. cumulative scores were calculated from ( a ). ( c ) H&E and Luxol fast blue (LFB) staining was performed same as in Fig. 1c . Depicted are typical pictures (magnification × 40) from EAE-induced PSA-treated WT or CD39 KO mice. All samples were collected ( n =4 sections per mouse, n =3 mice per group) at the peak of disease. Scale bars, 100 μm. ( d ) Tissues were collected at the onset of EAE and flow cytometric analysis of cells was performed. Mean±s.e.m. frequencies of activated subsets within total CD4 T cells were compared for the indicated sites ( n =4). ( e , f ) Total splenocytes were obtained from WT or CD39 KO mice treated as in a on day 14 of EAE induction and cultured in vitro with PSA, MOG 35–55 peptide, or a combination of both at escalating doses (10, 100 or 200 μg ml −1 of each). Supernatants were collected 48 h after culture. IL-10 ( e ) and IL-17A ( f ) were measured by ELISA. Mean±s.e.m. results are combined from two experiments ( n =3-4). ( g ) Rag KO recipient mice were reconstituted with splenic CD4 T cells from day 14 EAE-induced WT and CD39 KO mice treated with PSA as in a or PBS. Two weeks later, optimal active EAE was introduced into recipients. EAE was monitored till day 21. Mean±s.e.m. scores representative of two experiments are shown ( n =6–8, per group). * P <0.05; ** P <0.01. ( h ) Mean±s.e.m. cumulative scores were derived from g . P -value was calculated by Mann–Whitney U -test in a , b and h , by two-tailed Student’s t -test in d , e and f , and by Kruskal–Wallis test in g . Full size image To test whether CD39 differentially regulates pro- versus anti-inflammation cytokine responses to PSA or neural auto-antigen MOG 35–55 , splenocytes were isolated from PSA-treated, EAE-affected WT and CD39 KO mice, and recalled with dose-escalating PSA, MOG 35–55 peptide or combined in vitro for 48 h. IL-10 and IL-17A production was measured by enzyme-linked immunosorbent assay (ELISA). Although basal IL-10 release was comparable between WT and CD39 KO splenocytes, PSA dose-dependently increased IL-10 release from WT but not CD39 KO splenocytes. MOG 35–55 peptide suppressed IL-10 release from WT and CD39 KO splenocytes. Adding PSA to MOG 35–55 peptide restored dosage-dependent IL-10 release from WT splenocytes; IL-10 response of CD39 KO splenocytes remained compromised ( Fig. 5e ). In contrast, PSA decreased IL-17A release from WT splenocytes, whereas CD39 KO splenocytes displayed elevated IL-17A response when contrasted to WT splenocytes re-stimulated with dose-escalating PSA, MOG 35–55 peptide or combined in vitro ( Fig. 5f ). The requirement of CD39 in IL-10 responsiveness is antigen (PSA)-specific, as splenocytes from the same mice groups showed comparable in vitro IL-10 response to anti-CD3/CD28 beads ( Supplementary Fig. 12 ). Interferon-γ release, however, was only slightly enhanced in CD39 KO as opposed to WT splenocytes ( Supplementary Fig. 13 ). CD39 is also crucial for PSA-induced IL-10 release from CD4 T cells in vitro ( Supplementary Fig. 6D ). Thus, PSA-mediated reciprocal regulation of anti- versus pro-inflammatory cytokines is CD39-dependent. To determine whether CD4 T-cell-restricted CD39 signalling is required for PSA’s regulatory function during EAE, splenic CD4 T cells isolated from EAE-induced PSA- or PBS-treated WT or CD39 KO donor mice were introduced into Rag KO recipients, which lack mature B and T cells. Optimal active EAE was induced following reconstitution. As clinic curve revealed ( Fig. 5g ), the recipient group given PSA-modified WT CD4 T cells showed slower EAE progression. All groups culminated in comparable severity of EAE by day 21. Cumulative score quantified clinical differences ( Fig. 5h ). Rag KO recipients receiving naive WT or CD39 KO CD4 T cells were given the same regimen ( Supplementary Fig. 14 ). In both settings, CD4 T-cell-specific CD39 signalling is required for PSA-mediated control of EAE. In conclusion, TLR2 signalling is essential for PSA-mediated protection against CNS autoimmunity and localized expansion of CD39 + CD4 T cells defined as an indispensable regulatory subset both phenotypically and functionally. There exists a dynamic equilibrium in host-microbial mutualism. From the co-evolutionary perspective, both hosts and commensals must evolve regulatory mechanisms to quench deleterious mucosal and subsequent systemic inflammation. On the host side, several molecules have been discovered as the negative regulators of TLR-mediated inflammation such as the single immunoglobulin IL-1 receptor-related molecule, peroxisome proliferator-activated receptor-γ, nonspecific IgAs and inhibitory cytokines, for instance, IL-10 [38] , [39] . On the commensal side, B. fragilis capsular polysaccharide PSA typifies a molecular pattern that exploits TLR2 to deliver negative immune signals. The regulatory capacity of PSA could be due to its zwitterionic structure, as previous studies indicated that disruption of this structure inhibited PSA functions in vitro [40] . Multiple sclerosis is a CNS-targeting immune-mediated disease affected by both genetic and environmental factors. Murine EAE studies suggest that modification of intestinal commensals can alter disease outcomes [41] , [42] . The intestine is an important site for peripheral education of immune cells. Exposure to different commensal products may differentiate the CNS–antigen-reactive lymphocytes into an auto-aggressive or self-restrictive phenotype. Our previous studies identified that B. fragilis PSA could alleviate CNS inflammation [21] . We herein report that TLR2 is critical for PSA-mediated prevention of clinic progression, CNS demyelination and inflammation during EAE. TLR2 induced the tissue-specific expansion of a key regulatory CD39 + CD4 T-cell subset. Whether detection of PSA via antigen-presenting cell-restricted TLR2 is critical for CD4 + T cell acquisition of CD39 signal remains uncertain. It has been found that vesicle-associated PSA imposes specific genetic changes on DCs through TLR2 (ref. 24 ). Importantly, our previous studies indicated that CD103 + DCs accumulated at CLNs during PSA treatment of EAE and displayed elevated expression of TLR2 and major histocompatibility complex II [21] . Concomitant local expansion of both DC subsets and CD39 + CD4 T cells suggests that more than one pathway besides TLR2 may be involved in the process, which is currently under investigation. In this study, TLR2 liaised the connection between the commensal symbiosis factor PSA and CD39, a cell surface ectonucleotidase member of the ecto-nucleoside triphosphate diphosphohydrolase family. Extracellular ATP activates multiple immune functions that lead to inflammation [43] . Intestinal luminal contents comprise high concentrations of ATP produced by commensal bacteria. It has been reported that commensal-derived ATP is capable of inducing IL-6 and IL-23 production by lamina propria APCs and expands intestinal Th17 cells [44] . In this sense, B. fragilis PSA stimulation of CD39 signalling may represent a symbiont-evolved strategy to limit the excessive inflammatory response to commensal release of ATP. Indeed, we found that the selective induction of CD39 signalling on CD4 + T cell is required for PSA immune regulation at the systemic level. PSA seems more optimal in controlling Th17 than Th1 response, which is dependent on CD39 signalling. CD39 and CD73 coordinate hydrolysis of extracellular ATP to adenosine. The generated extracellular adenosine further inhibits T-cell-receptor-activated effector T cells via cognate A2a receptors [28] . Consistently, a reciprocal decrease of activated CD4 + T cells seems to accompany the increase of CD39 + CD4 T cells at CLNs during PSA treatment of EAE. CD39 is essential for the regulatory function of Foxp3 + CD4 Tregs [29] . It has been reported that CD39 + Foxp3 + CD4 Tregs but not CD39 − Foxp3 + CD4 Tregs can effectively suppress Th17 (ref. 45 ). However, several studies indicate that CD39 + CD4 T cell is in itself a regulatory subset regardless of Foxp3 (refs 46 , 47 ). It is speculated that CD39 + CD4 T cell consists of both Foxp3 + Tregs and Tr1 cells. Here we show that CD39 + CD4 T cell expressed remarkably higher IL-10 than CD39 − CD4 T cell. Moreover, CD39 is required for PSA-triggered IL-10 response. It is feasible that CD39 defines immuno-regulatory phenotype in both CD4 T cells and Foxp3 + CD4 Tregs. Previous studies showed that although PSA induced a limited quantitative increase of Foxp3 + CD4 Tregs, it robustly imprinted a functional suppressive genetic profile on Foxp3 + CD4 Tregs [20] . Therefore, CD39 is possibly the key signal that directs CD4 Tregs functional maturation in response to commensal antigen exposure. Collectively, this study on B.fragilis PSA deepens our understanding of the therapeutic potential and mechanism of commensal products in modulating CNS autoimmunity. Mice and treatment Eight-week-old female C57BL/6 mice were obtained from the Jackson Laboratories (Bar Harbor, ME). TLR2 KO mice were obtained from Dr Brent L. Berwin (Dartmouth College). IL-10 Thy1.1 reporter mice (10BiT) were obtained from Dr Casey T. Weaver (University of Alabama at Birmingham) and crossed with TLR2 KO strain by Yan Wang. CD39 KO mice were obtained from Dr Simon C. Robson (Harvard University). Rag-1, 2 DKO mice (Rag KO ) were obtained from Dr Mary Jo Turk (Dartmouth College). Mice were treated with 100 μg of purified B. fragilis PSA or PBS control by oral gavage every 3 days. Treatment begins 6 days before EAE induction and terminates 9 days after disease induction. All animal care and procedures were in accordance with protocols approved by the Institutional Animal Care and Use Committee of Dartmouth College. EAE induction Active optimal or sub-optimal EAE was induced with subcutaneous injection of 200 or 160 μg MOG 35–55 peptide (Peptides International; Louisville, KY), respectively, in 150 μl of Complete Freund’s Adjuvant (Sigma-Aldrich, St Louis, MO). On day 0 and 2 post immunization, intraperitoneal injection of 400 or 300 ng of Bordetella pertussis toxin (List Biological Laboratories, Campbell, CA) was, respectively, performed for optimal or sub-optimal EAE induction. For passive EAE in this study, Rag KO mice received intravenous injection of 3 × 10 6 purified splenic CD4 + T cells from indicated donors 2 weeks before active optimal EAE induction. EAE severity was scored daily using the standard scale. Histological analysis Transversal sections of spinal cords or brain stems were dissected from diseased animals and fixated with 10% formalin overnight. Paraffin-embedded samples were stained with H&E method for visualizing leukocyte infiltration or with Luxol fast blue method for assessing demyelination. Pathology Translational Research Division of Dartmouth-Hitchcock Medical Center performed all histology staining. Quantitative real-time PCR One microgram of mRNA was purified by QIAgen RNeasy kit (Qiagen, Germantown, MD) and reverse transcribed by MultiScribe Reverse Transcriptase (Invitrogen, Carlsbad, CA). Complementary DNA (200 ng) was amplified using SYBR Green PCR Master Mix (Applied Biosystems, Foster City, CA) on Bio-Rad CFX96 touch systems. The gene-specific primers are listed in Supplementary Table 1 . Relative gene expression (duplicates) were normalized to β-actin and calculated using the CT method, where relative expression=2 (exp–actin) × 1,000. Enzyme-linked immunosorbent assay Specific ELISA kits (Biolegend, San Diego, CA) were used to quantify cytokine levels in supernatants. Cells were cultured in 96-well or 48-well tissue plates at 2 × 10 6 cells per ml concentration in the presence of indicated soluble reagents or anti-CD3/CD28 Dynabeads (Invitrogen, Carlsbad, CA) for 48 h and supernatants were collected. Flow cytometric analysis Singe cell preparations were isolated from indicated tissue sites and flow stained. Fluorochrome-conjugated monoclonal antibodies specific to mouse CD4 (clone GK1.5), CD19 (clone 6D5), CD25 (clone PC61.5), CD29 (clone HMβ1-1), CD39 (clone 24DMS1), CD40L (clone MR1), CD44 (clone IM7), CD49d (clone R1-2), CD62L (clone MEL-14), CD69 (clone H1.2F3), CD73 (Clone eBioTY/11.8), CD103 (clone 2E7), CD127 (clone A7R34), 4-1BB (clone 17B5), GITR (clone DTA-1), ICOS (clone 7E.17G9), LAG-3 (clone eBioC9B7W), latency-associated peptide (clone TW7-16B4), PD-1 (clone 29F.1A12) and Thy1.1 (clone OX-7) (1:400 dilution, Biolegend or eBioscience) were used in various combinations for cell surface staining. Biotin-labelled anti-VISTA monoclonal antibody was provided by Dr Li Wang (Medical College of Wisconsin). The Fc receptor was blocked by CD16/32 antibody (Biolegend). For Foxp3 (1:400 dilution; clone FJK-16 s, eBioscience) and CTLA-4 (1:400 dilution; clone UC10-4B9, Biolegend), cells were treated by eBioscience intracellular fixation/permeabilization buffer set and intracellular staining was performed. Stained cells were assayed by MACSQuant Analyzers (Miltenyi, Bergisch Gladbach, Germany). Cell purifications Splenic CD4 + T cells were enriched with mouse CD4 + T-cell isolation kit (StemCell Technologies, Vancouver, Canada) according to provided protocols. Statistical analysis Two-tailed Student’s t -test was used to show statistical differences of mRNA relative expression in quantitative RT–PCR, fluorescence intensity or cell frequencies in FACS and cytokine levels in ELISA. Analysis of variance followed by post-hoc t -test was used where applicable. Mann–Whitney U -test was applied to cumulative clinic scores. Kruskal–Wallis test was applied when multiple groups of clinic curves were compared. Data are shown as means±s.e.m. P -values <0.05, <0.01 and <0.001 were indicated. How to cite this article: Wang, Y. et al . An intestinal commensal symbiosis factor controls neuroinflammation via TLR2-mediated CD39 signalling. Nat. Commun. 5:4432 doi: 10.1038/ncomms5432 (2014).